KaiC intersubunit communication facilitates robustness of circadian rhythms in cyanobacteria The cyanobacterial circadian clock is the only model clock to have been reconstituted in vitro . KaiC, the central clock component, is a homohexameric ATPase with autokinase and autophosphatase activities. Changes in phosphorylation state have been proposed to switch KaiC’s activity between autokinase and autophosphatase. Here we analyse the molecular mechanism underlying the regulation of KaiC’s activity, in the context of its hexameric structure. We reconstitute KaiC hexamers containing different variant protomers, and measure their autophosphatase and autokinase activities. We identify two types of regulatory mechanisms with distinct functions. First, local interactions between adjacent phosphorylation sites regulate KaiC’s activities, coupling the ATPase and nucleotide-binding states at subunit interfaces of the CII domain. Second, the phosphorylation states of the protomers affect the overall activity of KaiC hexamers via intersubunit communication. Our findings indicate that intra-hexameric interactions play an important role in sustaining robust circadian rhythmicity. Circadian rhythms, endogenous oscillations with periods of ~24 h, are found in many organisms, and they enhance fitness in an alternating day/night environment [1] . Cyanobacteria are the simplest organisms that exhibit circadian rhythms [2] . Three clock genes, kaiA , kaiB and kaiC , are essential components of the timekeeping apparatus of the cyanobacterium Synechococcus elongatus PCC 7942 (hereafter, Synechococcus ) [3] . To date, the cyanobacterial clock is the sole circadian system to have been reconstituted in vitro ; in a system using purified proteins, the phosphorylation state of KaiC exhibits robust circadian rhythms generated by interactions of KaiA and KaiB in the presence of ATP [4] , [5] . The simplicity of the cyanobacterial in vitro system makes it ideal for understanding the principles underlying circadian clocks. KaiC, the central component of the system, is a double-domain P-loop ATPase consisting of N-terminal CI and C-terminal CII domains, each of which contains ATPase motifs [3] , [6] , [7] , [8] . In addition to ATPase activity, KaiC has autokinase and autophosphatase activities [9] , [10] , [11] . KaiA enhances KaiC phosphorylation, whereas KaiB inhibits the effects of KaiA [6] , [10] , [11] , [12] . KaiC has two adjacent phosphorylation sites at serine 431 (S431) and threonine 432 (T432) in the CII domain [13] . During each circadian cycle, phosphorylation of KaiC proceeds in an ordered pattern. Unphosphorylated KaiC (S/T) is first phosphorylated at T432 (S/pT), which is further phosphorylated to the double-phosphorylated form (pS/pT). The T432 residue of pS/pT is dephosphorylated first, yielding KaiC phosphorylated only at S431 (pS/T). Phosphorylation of KaiC is modulated by the phosphorylation state of KaiC itself and by KaiC’s phosphorylation state-dependent interactions with KaiA and KaiB. KaiA stimulates KaiC phosphorylation by repeated association with KaiC, whereas KaiB preferentially binds pS/T, which forms a ternary complex with KaiA and inactivates it. These regulatory interactions are thought to be basis of the ordered phosphorylation cycle of KaiC [14] , [15] . KaiC is a homohexameric enzyme of the RecA/DnaB superfamily [16] , [17] , [18] . Several studies have indicated that cooperative regulation of ATPase activity in hexameric ATPases is important for their biological functions [19] , [20] , [21] , [22] , [23] , [24] . Furthermore, several studies have proposed mathematical models of robust oscillation of KaiC phosphorylation, based on the hexameric structure of KaiC [25] , [26] , [27] , [28] , [29] , [30] , [31] , [32] , [33] . The crystal structures of Synechococcus KaiC show that ATP molecules bind at each subunit interface [17] , the autophosphorylation sites face the ATP molecules on the neighbouring protomers [34] and the putative catalytic glutamates of the ATPase motif are at the subunit interface [17] , [34] . KaiC mutants in which the nucleotide-binding site is altered are kinase-deficient [35] , [36] . Furthermore, a previous study, using thermophilic cyanobacterium Thermosynechococcus elongatus BP-1, demonstrated that phosphorylation occurs at the subunit interfaces of KaiC [37] . These results suggest that KaiC’s three activities (ATPase, autokinase and autophosphatase), which are essential for circadian rhythm, are coupled and regulated at subunit interfaces. It has been assumed that the KaiC’s regulatory mechanisms as hexamer are crucial for the circadian clock; however, the mechanism of how phosphorylation states regulate kinase/phosphatase activities at subunit interfaces and how ATPase activity is coupled to kinase/phosphatase activity has been unclear. In addition, the functional importance of the hexameric structure in determining circadian rhythm has not been experimentally demonstrated. Recently, we demonstrated the dissociation of Synechococcus KaiC hexamers into monomers and the reconstitution of functional hexamers [38] . This method has made possible mutant mixing experiments to analyse interactions between KaiC’s activities at subunit interface. In this study, to elucidate the regulation of KaiC’s activities by its phosphorylation state in the context of its hexameric structure, we prepare hexamers containing various combinations of wild-type (WT) protein or mutants in the phosphorylation site or ATPase catalytic site, and analyse these hexamers in autodephosphorylation and autophosphorylation assays. We identify two types of regulatory mechanisms. First, the phosphorylation state of one phosphorylation site locally affects its own subunit interfaces in a manner that influences phosphorylation of the adjacent residue, coupling the ATPase and nucleotide-binding state of the CII domain. Second, the phosphorylation states of protomers affect the global activity of the KaiC hexamer via intersubunit interactions. Our results reveal the molecular mechanism underlying the autoregulation of KaiC’s activity, by which KaiC’s autokinase and autophosphatase activities are regulated by its phosphorylation state. Furthermore, our data provide unexpected evidence for intersubunit communication within KaiC hexamers. The observations suggest that intersubunit communication precisely synchronizes KaiC subunits to avoid dephasing and facilitates robustness of circadian rhythms in cyanobacteria. Preparation of hexamers with altered subunit interfaces To elucidate the regulatory mechanism of KaiC’s activities in the context of the hexameric structure, we prepared hexamers containing variants protomers by mixing KaiC mutants. As Synechococcus KaiC exists as a hexamer [39] , we first dissociated hexamers into monomers by removing ATP, and then reconstituted hexamers by mixing equal amounts of KaiC-variant monomers in the presence of ATP. After monomerization and reconstitution, KaiC-WT hexamers exhibited normal phosphorylation rhythm ( Supplementary Fig. S1 ), indicating that the monomerization/reconstitution process did not affect KaiC function, as shown previously [38] . To test whether phosphorylation occurs at the subunit interfaces, we mixed two mutants: KaiC-AA, in which both phosphorylation sites were replaced with alanine, and KaiC-E318Q, in which the putative catalytic glutamate of the ATPase motif was replaced with glutamine. The phosphorylation sites face E318 across the ATP molecules at the subunit interface ( Supplementary Fig. S2 ; refs 17 , 34 ). Individually, both mutants exhibit very low or no phosphorylation [36] , [37] , [40] ; however, mixed hexamers are expected to have mosaic subunit interfaces, including some intact interfaces and should therefore undergo phosphorylation if the hypothesis regarding the location of phosphorylation is correct ( Fig. 1a ). To characterize hexamer composition, a FLAG-tag and His-tag were added to KaiC-E318Q and KaiC-AA, respectively. Reconstituted hexamers (R) were subjected to immunoprecipitation with anti-FLAG antibody; both His-tagged KaiC-AA and FLAG-tagged KaiC-E318Q were detected in eluates ( Fig. 1c ; Supplementary Fig. S3 ), indicating that KaiC-AA and KaiC-E318Q monomers interacted to form mixed hexamers. About 50% of the monomers in reconstituted hexamers were KaiC-E318Q ( Fig. 1c ), confirming that the reconstitution procedures yielded mixed hexamers in which the two mutant subunits were present in 1:1 stoichiometry. We also confirmed that hexamers did not spontaneously exchange protomers within 30 min after mixing ( Fig. 1c ). 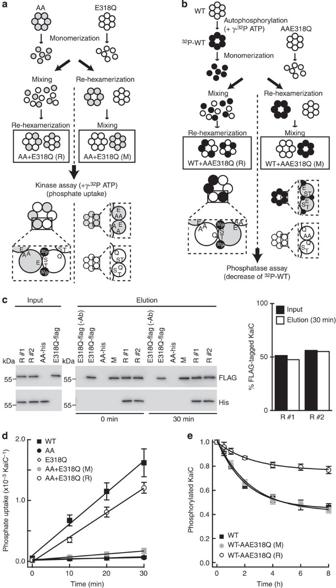Figure 1: KaiC autodephosphorylation and autophosphorylation occur at subunit interfaces within KaiC hexamers. (a) Schematic representation of procedures forFig. 1d. Hexamers were reconstituted by mixing equal amounts of monomers (AA+E318Q [R]). The mixtures of hexamers (AA+E318Q [M]) were prepared from KaiC-AA and KaiC-E318Q hexamers. (b) Schematic representation of procedures forFig. 1e. KaiC-WT was labelled with [γ-32P] ATP and dissociated into monomers. Equal amounts of32P-labelled KaiC-WT and KaiC-AAE318Q monomers were mixed to prepare reconstituted mixed hexamers (WT+AAE318Q [R]). KaiC-WT and KaiC-AAE318Q hexamers were mixed to prepare the mixture of hexamers (WT+AAE318Q [M]). (c) Characterization of hexamer composition. Reconstituted hexamers from FLAG-tagged KaiC-E318Q and His-tagged KaiC-AA monomers (R) and a mixture of hexamers (M) were analysed by immunoprecipitation and the percentage of FLAG-tagged KaiC-E318Q in reconstituted hexamers was estimated. Data were collected from two independent preparations of reconstituted hexamers (R#1 and R#2). (d) Kinase activity determined by phosphate-uptake assay of KaiC-WT (closed squares); KaiC-AA (closed circles); KaiC-E318Q (open diamonds); a mixture of KaiC-AA and KaiC-E318Q hexamers (AA+E318Q [M]; closed grey circles) and reconstituted hexamers from a mixture of KaiC-AA and KaiC-E318Q monomers (AA+E318Q [R]; open circles). Data are presented as means±s.e.m. (n=4). Solid line shows the linear fit to the data, yielding a rate constant of 0.0519, min−1±0.00254 for WT, 0.0403, min−1±0.00174 for AA+E318Q (R), 0.005 min−1±9.87 × 10−19for AA+E318Q (M), 0.002 min−1±0.000316 for E318Q and 0.001 min−1±1.23 × 10−19for AA. (e) Dephosphorylation of KaiC-WT in KaiC-WT (closed squares), a mixture of KaiC-WT and KaiC-AAE318Q hexamers (WT+AAE318Q [M]; closed grey circles) and reconstituted hexamers from a mixture of KaiC-WT and KaiC-AAE318Q monomers (WT+AAE318Q [R]; open circles). Phosphatase activity was determined by monitoring the decrease in intensity of the32P-labelled band. Data were normalized to the level of phosphorylated KaiC at 0 h, and are presented as means±s.d. (n=4). The first-order rate constants were obtained by single exponential curve fit (solid line): 0.48193, h−1±0.0515 for WT, 0.41913, h−1±0.0577 for WT+AAE318Q (M) and 0.39143, h−1±0.0257 for WT+AAE318Q (R). Figure 1: KaiC autodephosphorylation and autophosphorylation occur at subunit interfaces within KaiC hexamers. ( a ) Schematic representation of procedures for Fig. 1d . Hexamers were reconstituted by mixing equal amounts of monomers (AA+E318Q [R]). The mixtures of hexamers (AA+E318Q [M]) were prepared from KaiC-AA and KaiC-E318Q hexamers. ( b ) Schematic representation of procedures for Fig. 1e . KaiC-WT was labelled with [γ- 32 P] ATP and dissociated into monomers. Equal amounts of 32 P-labelled KaiC-WT and KaiC-AAE318Q monomers were mixed to prepare reconstituted mixed hexamers (WT+AAE318Q [R]). KaiC-WT and KaiC-AAE318Q hexamers were mixed to prepare the mixture of hexamers (WT+AAE318Q [M]). ( c ) Characterization of hexamer composition. Reconstituted hexamers from FLAG-tagged KaiC-E318Q and His-tagged KaiC-AA monomers (R) and a mixture of hexamers (M) were analysed by immunoprecipitation and the percentage of FLAG-tagged KaiC-E318Q in reconstituted hexamers was estimated. Data were collected from two independent preparations of reconstituted hexamers (R#1 and R#2). ( d ) Kinase activity determined by phosphate-uptake assay of KaiC-WT (closed squares); KaiC-AA (closed circles); KaiC-E318Q (open diamonds); a mixture of KaiC-AA and KaiC-E318Q hexamers (AA+E318Q [M]; closed grey circles) and reconstituted hexamers from a mixture of KaiC-AA and KaiC-E318Q monomers (AA+E318Q [R]; open circles). Data are presented as means±s.e.m. ( n =4). Solid line shows the linear fit to the data, yielding a rate constant of 0.0519, min −1 ±0.00254 for WT, 0.0403, min −1 ±0.00174 for AA+E318Q (R), 0.005 min −1 ±9.87 × 10 −19 for AA+E318Q (M), 0.002 min −1 ±0.000316 for E318Q and 0.001 min −1 ±1.23 × 10 −19 for AA. ( e ) Dephosphorylation of KaiC-WT in KaiC-WT (closed squares), a mixture of KaiC-WT and KaiC-AAE318Q hexamers (WT+AAE318Q [M]; closed grey circles) and reconstituted hexamers from a mixture of KaiC-WT and KaiC-AAE318Q monomers (WT+AAE318Q [R]; open circles). Phosphatase activity was determined by monitoring the decrease in intensity of the 32 P-labelled band. Data were normalized to the level of phosphorylated KaiC at 0 h, and are presented as means±s.d. ( n =4). The first-order rate constants were obtained by single exponential curve fit (solid line): 0.48193, h −1 ±0.0515 for WT, 0.41913, h −1 ±0.0577 for WT+AAE318Q (M) and 0.39143, h −1 ±0.0257 for WT+AAE318Q (R). Full size image Phosphorylation reactions are regulated at subunit interfaces We performed autokinase assays using reconstituted (R) mixed hexamers (AA+E318Q [R]), and found that they exhibited phosphate-incorporation activity equal to or greater than that of KaiC-WT hexamers, after adjusting for the fact that the number of intact phosphorylation sites in AA+E318Q (R) was half of that in WT hexamers. By contrast, KaiC-AA alone did not incorporate 32 P, and KaiC-E318Q alone or in mixtures (M) of hexameric KaiC-AA and KaiC-E318Q (AA+E318Q [M]) exhibited only slight kinase activity ( Fig. 1d and Supplementary Fig. S4 ). We then prepared hexamers from a mixture of 32 P-labelled WT and unlabelled KaiC-AAE318Q monomers (that is, KaiC monomers containing both the AA and E318Q mutations) to determine whether this mixing would alter phosphatase activity ( Fig. 1b ). KaiC-WT underwent dephosphorylation, as revealed by a decrease in the level of 32 P-labelled KaiC; however, the level of 32 P-labelled KaiC-WT stabilized in reconstituted mixed hexamers (WT+AAE318Q [R]). The interfaces between WT and AAE318Q protomers are predicted to be stuck in the phosphorylated state, because protomers with the E318Q mutation should inhibit dephosphorylation of the neighbouring KaiC-WT protomers. There was no difference in phosphatase activity between KaiC-WT hexamers and a mixture of WT and AAE318Q hexamers (WT+AAE318Q [M]) ( Fig. 1e and Supplementary Fig. S4 ). These data suggest that the kinase and phosphatase activities occur at subunit interfaces. KaiC’s activities are related to nucleotide-binding states The results of Fig. 1 showed that the putative catalytic glutamate residue (E318) is important for both autokinase and autophosphatase activities. KaiC consists of CI and CII domains, each of which contains ATPase motifs ( Fig. 2a ; refs 3 , 6 , 7 , 8 ). We investigated the relationship between the ATPase activity of the CI and CII domains and autokinase/autophosphatase activity, using mutants containing mutations in the putative catalytic glutamate residues in either CI or CII domain (KaiC-E77QE78Q and KaiC-E318Q). Although we tried to prepare KaiC-E318QE319Q, we could not purify this protein because it became insoluble during preparation. ATPase activity of KaiC-E77QE78Q was ~50% of the KaiC-WT activity, confirming that these resides are responsible for the ATPase activity of CI domain ( Fig. 2b ). ATPase activity of KaiC-AA was higher than that of the KaiC-WT ( Fig. 2b ; refs 7 , 8 ). The elevated activity in KaiC-AA is thought to originate from CII domain, because the ATPase activity of the CI domain is not affected by phosphorylation state [8] . Although the ATPase activity of the KaiC-E318Q mutant was similar to that of KaiC-WT, the E318Q mutation decreased the elevated activity of KaiC-AA ( Fig. 2b ). Therefore, we concluded that E318 is responsible for the ATPase activity of CII domain. 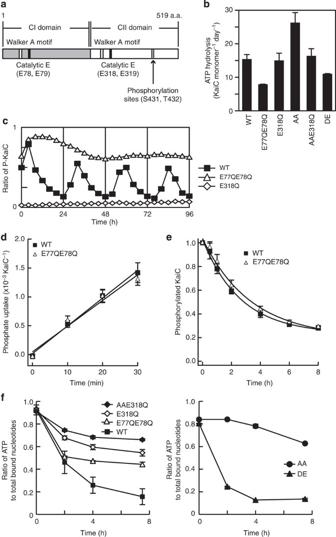Figure 2: ATPase activity and nucleotide-binding states of the CII domain regulate phosphorylation and dephosphorylation. (a) Schematic illustrations of tandem duplicated domains of KaiC, N-terminal CI and C-terminal CII. Locations of P loops, catalytic carboxylates and two phosphorylation sites are indicated. (b) ATPase activity of WT and mutant KaiC. Data are presented as means±s.d. (n=3–6). (c) Quantitation of phosphorylation of KaiC-WT (closed square), KaiC-E77QE78Q (open triangle) and KaiC-E318Q (open diamond) in the presence of KaiA and KaiB. The ratio of phosphorylated KaiC to total KaiC is plotted. (d) Kinase activity of KaiC-WT (closed square) and KaiC-E77QE78Q (open triangle) were determined by phosphate-uptake assay. Data are presented as means±s.e.m. (n=4). Solid lines show the linear fit to the data, giving a rate constant of 0.0481, min−1±0.00238 for WT and 0.0444, min−1±0.00541 for E77QE78Q. (e) Dephosphorylation of KaiC-WT (closed square) and KaiC-E77QE78Q (open triangle). KaiC was autophosphorylated with [γ-32P]ATP, then allowed to dephosphorylate. Following SDS–PAGE,32P-labelled KaiC was detected by autoradiography. Phosphatase activity was determined by monitoring the decrease in intensity of the32P-label band. Data were normalized to the level of phosphorylated KaiC at 0 h, and are presented as means±s.d. (n=4). The first-order rate constants were obtained by single exponential curve fit (solid line): 0.37864, h−1±0.0474 for WT and 0.30081, h−1±0.0535 for E77QE78Q. (f) Characterization and quantification of KaiC-bound nucleotides. KaiC hexamers were reconstituted from monomers in the presence of [α-32P]ATP, and the samples were incubated at 30 °C. The ratio of ATP relative to total nucleotides bound to KaiC-WT (closed squares), KaiC-E77QE78Q (open triangle), KaiC-E318Q (open diamonds), KaiC-AAE318Q (closed diamonds), KaiC-AA (closed circles) or KaiC-DE (closed triangles) was plotted against time. Data represent means±s.d. (n=4). Figure 2: ATPase activity and nucleotide-binding states of the CII domain regulate phosphorylation and dephosphorylation. ( a ) Schematic illustrations of tandem duplicated domains of KaiC, N-terminal CI and C-terminal CII. Locations of P loops, catalytic carboxylates and two phosphorylation sites are indicated. ( b ) ATPase activity of WT and mutant KaiC. Data are presented as means±s.d. ( n =3–6). ( c ) Quantitation of phosphorylation of KaiC-WT (closed square), KaiC-E77QE78Q (open triangle) and KaiC-E318Q (open diamond) in the presence of KaiA and KaiB. The ratio of phosphorylated KaiC to total KaiC is plotted. ( d ) Kinase activity of KaiC-WT (closed square) and KaiC-E77QE78Q (open triangle) were determined by phosphate-uptake assay. Data are presented as means±s.e.m. ( n =4). Solid lines show the linear fit to the data, giving a rate constant of 0.0481, min −1 ±0.00238 for WT and 0.0444, min −1 ±0.00541 for E77QE78Q. ( e ) Dephosphorylation of KaiC-WT (closed square) and KaiC-E77QE78Q (open triangle). KaiC was autophosphorylated with [γ- 32 P]ATP, then allowed to dephosphorylate. Following SDS–PAGE, 32 P-labelled KaiC was detected by autoradiography. Phosphatase activity was determined by monitoring the decrease in intensity of the 32 P-label band. Data were normalized to the level of phosphorylated KaiC at 0 h, and are presented as means±s.d. ( n =4). The first-order rate constants were obtained by single exponential curve fit (solid line): 0.37864, h −1 ±0.0474 for WT and 0.30081, h −1 ±0.0535 for E77QE78Q. ( f ) Characterization and quantification of KaiC-bound nucleotides. KaiC hexamers were reconstituted from monomers in the presence of [α- 32 P]ATP, and the samples were incubated at 30 °C. The ratio of ATP relative to total nucleotides bound to KaiC-WT (closed squares), KaiC-E77QE78Q (open triangle), KaiC-E318Q (open diamonds), KaiC-AAE318Q (closed diamonds), KaiC-AA (closed circles) or KaiC-DE (closed triangles) was plotted against time. Data represent means±s.d. ( n =4). Full size image The E318Q mutation inhibited both autokinase and autophosphatase activities ( Fig. 1 ), and KaiC-E318Q was constitutively dephosphorylated even in the presence of KaiA and KaiB ( Fig. 2c ). By contrast, phosphatase and kinase activities did not differ between KaiC-WT and KaiC-E77QE78Q ( Fig. 2d,e , Supplementary Fig. S4 ). As the dephosphorylation process requires ADP as a phosphate acceptor [38] , we next examined the time-dependent changes in the levels of nucleotides bound to KaiC. In KaiC-WT, the ratio of ADP to total bound nucleotides increased to 0.8 after 8 h of incubation. Although it is not possible to accurately determine whether ADPs bind on CI or CII, a previous study suggested that the CII domain is responsible for ADP binding to KaiC, because CII-truncated KaiC binds only ATP [38] . We found that KaiC-AAE318Q, which was defected with phosphatase, was predominantly present in the ATP-bound form, indicating that the CII domain is in the ATP-bound form in KaiC-AAE318Q ( Fig. 2f ). By contrast, 50% of the nucleotides that bound to KaiC-E77QE78Q, which had phosphatase activity similar to KaiC-WT, were ATP. This observation indicated that the CI domain was in the ATP-bound form, and CII domain was in the ADP-bound form in KaiC-E77QE78Q as with CII domain in KaiC-WT ( Fig. 2f ). Taken together, these data indicate that steady-state ADP binding by the CII domain is correlated with normal phosphatase activity. Furthermore, we found that the phosphorylation states also modulated nucleotide-binding state: KaiC-AA was predominantly in the ATP-bound form, whereas KaiC-DE was predominantly in the ADP-bound form ( Fig. 2f ). These data indicated that the interface between two CII-domain subunits is the fundamental reaction unit for both phosphorylation and dephosphorylation. Furthermore, autokinase and autophosphatase activities were closely related to ATPase activity and the nucleotide-binding state of the CII domain. Hexameric composition influences KaiC activity The balance between autokinase and autophosphatase activities of KaiC swings back and forth on a circadian cycle, modulated by KaiC phosphorylation states and KaiC’s phosphorylation state-dependent interactions with KaiA and KaiB ( Supplementary Fig. S5 ; refs 14 , 15 ). These modes of regulation are thought to be crucial for the ordered phosphorylation cycle. Based on the results shown in Figs 1 and 2 , it is likely that each site’s phosphorylation state affects the interactions of its own subunit interface with regard to ATPase activity and the nucleotide-binding state of the CII domain, and thereby influences phosphorylation of the adjacent residue. Alternatively, protomer phosphorylation states might affect the overall activity of KaiC hexamers via intersubunit interactions. During the phosphorylation phase, hexamers are enriched in S/pT, whereas pS/T predominates in the dephosphorylation phase; however, the phosphorylation states of protomers within a hexamer are non-uniform ( Fig. 3a ; refs 14 , 15 ). Thus, a pT- or pS-protomer might affect the activity of other protomers in the same hexamer. 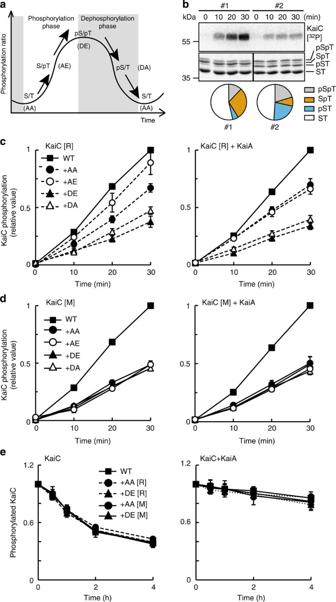Figure 3: The combination of phosphorylation states in the KaiC hexamer alters the kinase activity of KaiC. (a) Schematic of the ordered KaiC phosphorylation cycle and amino-acid substitutions that mimic each phosphorylation state. (b) Autokinase activity (#1, KaiC enriched in pT; #2, KaiC enriched in pS) was determined by phosphate-uptake assay. Upper: autoradiograph of32P-labelled KaiC. Lower: coomassie brilliant blue-stained gel. Four bands with different mobilities were detected. From most to least mobile, bands represent the S/T, pS/T, S/pT and pS/pT forms of KaiC14. Pie charts show the distribution of phosphorylation states at time zero. (c) The autokinase assay was performed using reconstituted hexamers in the absence (left) or presence (right) of KaiA. Phosphorylation is shown for KaiC-WT (closed squares); mixed hexamers of KaiC-WT and KaiC-AA (closed circles); KaiC-WT and KaiC-AE (open circles); KaiC-WT and KaiC-DE (closed triangles); and KaiC-WT and KaiC-DA (open triangle). Data were normalized against the maximum signal obtained. Data are presented as means±s.e.m. (n=7). (d) Equal amounts of KaiC-WT and mutant KaiC hexamers were mixed, and the kinase activity was measured in the absence (left) or presence (right) of KaiA. Phosphorylation is shown for KaiC-WT (closed squares) and KaiC-WT mixed with KaiC-AA (closed circles), KaiC-AE (open circles), KaiC-DE (closed triangles) or KaiC-DA (open triangles). Data were normalized against the maximum signal obtained. Data are presented as means±s.e.m. (n=7). (e) Measurement of phosphatase activity in the absence (left) or presence (right) of KaiA. Hexamer was reconstituted with32P-labelled KaiC-WT and non-labelled KaiC-AA or KaiC-DE monomers. Levels of32P-labelled KaiC-WT were measured by autoradiography in KaiC-WT (closed squares and solid line); mixed hexamers of KaiC-WT and KaiC-AA (closed circles and dashed line); a mixture of KaiC-WT and KaiC-AA hexamers (closed circles and solid line); mixed hexamers of KaiC-WT and KaiC-DE (closed triangles and dashed line); a mixture of KaiC-WT and KaiC-DE hexamers (closed triangles and solid line). ‘M’ indicates a mixture of hexamers and ‘R’ indicates a reconstituted hexamer. Data were normalized to the level of phosphorylated KaiC at 0 h (defined as 1). Data are presented as means±s.d. (n=5). Figure 3: The combination of phosphorylation states in the KaiC hexamer alters the kinase activity of KaiC. ( a ) Schematic of the ordered KaiC phosphorylation cycle and amino-acid substitutions that mimic each phosphorylation state. ( b ) Autokinase activity (#1, KaiC enriched in pT; #2, KaiC enriched in pS) was determined by phosphate-uptake assay. Upper: autoradiograph of 32 P-labelled KaiC. Lower: coomassie brilliant blue-stained gel. Four bands with different mobilities were detected. From most to least mobile, bands represent the S/T, pS/T, S/pT and pS/pT forms of KaiC [14] . Pie charts show the distribution of phosphorylation states at time zero. ( c ) The autokinase assay was performed using reconstituted hexamers in the absence (left) or presence (right) of KaiA. Phosphorylation is shown for KaiC-WT (closed squares); mixed hexamers of KaiC-WT and KaiC-AA (closed circles); KaiC-WT and KaiC-AE (open circles); KaiC-WT and KaiC-DE (closed triangles); and KaiC-WT and KaiC-DA (open triangle). Data were normalized against the maximum signal obtained. Data are presented as means±s.e.m. ( n =7). ( d ) Equal amounts of KaiC-WT and mutant KaiC hexamers were mixed, and the kinase activity was measured in the absence (left) or presence (right) of KaiA. Phosphorylation is shown for KaiC-WT (closed squares) and KaiC-WT mixed with KaiC-AA (closed circles), KaiC-AE (open circles), KaiC-DE (closed triangles) or KaiC-DA (open triangles). Data were normalized against the maximum signal obtained. Data are presented as means±s.e.m. ( n =7). ( e ) Measurement of phosphatase activity in the absence (left) or presence (right) of KaiA. Hexamer was reconstituted with 32 P-labelled KaiC-WT and non-labelled KaiC-AA or KaiC-DE monomers. Levels of 32 P-labelled KaiC-WT were measured by autoradiography in KaiC-WT (closed squares and solid line); mixed hexamers of KaiC-WT and KaiC-AA (closed circles and dashed line); a mixture of KaiC-WT and KaiC-AA hexamers (closed circles and solid line); mixed hexamers of KaiC-WT and KaiC-DE (closed triangles and dashed line); a mixture of KaiC-WT and KaiC-DE hexamers (closed triangles and solid line). ‘M’ indicates a mixture of hexamers and ‘R’ indicates a reconstituted hexamer. Data were normalized to the level of phosphorylated KaiC at 0 h (defined as 1). Data are presented as means±s.d. ( n =5). Full size image To test this hypothesis, we examined S/pT-enriched or pS/T-enriched KaiC’s activity. When KaiC was incubated at 4 or 30 °C in the absence of KaiA, KaiC tended toward the phosphorylated or dephosphorylated state, respectively ( Supplementary Fig. S6 ; refs 41 , 42 ). At 4 °C, KaiC had lower autophosphatase activity and higher phosphate-uptake activity than at 30 °C. We also found that KaiC at 4 °C predominantly existed in the ATP-bound form ( Supplementary Fig. S6 ). These data reveal that phosphorylation state is temperature-dependent. By changing the incubation temperature, we could prepare S/pT-enriched or pS/T-enriched KaiC, corresponding to the phosphorylation or dephosphorylation phase, respectively. The resultant samples contained mixtures of molecules, each of which had different phosphorylation states: the percentages of pS/T, S/pT and pS/pT were altered by varying the preparation method, and ~50% of KaiC molecules were unphosphorylated ( Fig. 3b ). The S/pT-enriched KaiC exhibited higher phosphate-uptake activity than pS/T-enriched KaiC, either in the absence ( Fig. 3b ; Supplementary Fig. S3 ) or presence ( Supplementary Fig. S7 ) of KaiA. As the kinase activities may have been underestimated due to ongoing phosphatase activity, higher amounts of 32 P make it possible to detect higher kinase activity or lower phosphatase activity. These results showed that the hexameric composition of phosphorylation states influences autokinase/autophosphatase activity, suggesting the existence of intersubunit interactions. Intersubunit interactions control autokinase activity To further analyse intra-hexameric interaction, we prepared reconstituted hexamers from 1:1 mixtures of KaiC-WT and phosphorylation-mutant monomers, using the same procedure as for the experiments shown in Fig. 1 ( Supplementary Fig. S8 ). In reconstituted mixed hexamers (R), the subunit interface of the phosphorylation site of KaiC-WT is normal; however, the number of intact reaction units will be halved because half of the protomers will be fixed in a specific phosphorylated state and therefore unable to incorporate phosphate. Therefore, if kinase activity is regulated locally at reaction units, global activity should be half that of KaiC-WT. Alternatively, if there are intersubunit interactions, kinase activity will change depending on the phosphorylation state of the mixed mutant. We prepared four mutants, KaiC-AA, -AE, -DE and -DA, which mimic phosphorylation states in the KaiC phosphorylation cycle ( Fig. 3a ). To characterize hexamer composition, a FLAG-tag and His-tag were added to KaiC-WT and KaiC-mutant, respectively. We confirmed that KaiC-WT and KaiC-mutant monomers interacted and formed random mixed hexamers in an approximately 1:1 ratio ( Supplementary Fig. S9 ). KaiA enhanced kinase activity and inhibited phosphatase activity; however, KaiB only inhibited the effect of KaiA under specific phosphorylation states of KaiC ( Supplementary Fig. S5 ; refs 6 , 10 , 11 , 12 ). We observed phosphate incorporation in the absence or presence of KaiA ( Fig. 3c ). All radiolabeled signals were the result of KaiC-WT phosphorylation, because the mutant proteins cannot incorporate phosphate ( Supplementary Fig. S10 ). The observed kinase activity was dependent on the specific combination of WT and mutant proteins. The kinase activity of KaiC-WT was affected negatively by the presence of KaiC-DE and -DA. By contrast, KaiC-AA and -AE had positive effects on the kinase activity of KaiC-WT subunits ( Fig. 3c ). We confirmed that there were no significant changes in protein levels over the course of the assay ( Supplementary Fig. S10 ). In the presence of KaiA, the kinase activity of KaiC-WT was decreased by KaiC-DE and -DA and increased by KaiC-AA and -AE, similar to the results obtained with KaiC alone ( Fig. 3c ). By contrast, the incorporation of phosphate in the mixture of WT and mutant hexamers (M) was half that of pure KaiC-WT, because the total concentration of KaiC-WT in the reaction mixture was halved ( Fig. 3d ). These observations provide further confirmation that there were no interactions between hexamers. Phosphatase activity is regulated at the subunit interface Using the same strategies, we investigated intersubunit interactions during the dephosphorylation. KaiC-WT underwent dephosphorylation similarly under all conditions ( Fig. 3e and Supplementary Fig. S11 ). The presence of KaiC-AA or KaiC-DE had no effect on the dephosphorylation of KaiC-WT. Thus, regulation of phosphatase activity by phosphorylation state ( Supplementary Fig. S5 ) may occur only at reaction units composed of subunit interfaces. The kinase activities may have been underestimated as mentioned above; however, phosphatase activity was not affected by the specific combination of WT and mutant proteins ( Fig. 3e ), so we consider the differences in Fig. 3c to reflect altered kinase activity. These results suggest that kinase activity is regulated by intersubunit interactions within hexamers. Intersubunit interaction is important for robust rhythms To determine whether intersubunit interactions are important for circadian rhythms, we incubated reconstituted (R) mixed hexamers prepared as in Fig. 3 in the presence of KaiA and KaiB, and monitored the phosphorylation states of KaiC-WT. The rhythmic change in KaiC-WT phosphorylation was not observed for all 1:1 mixtures of WT and mutant protein ( Fig. 4a ). KaiC-WT was phosphorylated when combined with KaiC-AA or -AE subunits, which increased the kinase activity of KaiC-WT, whereas KaiC-WT was dephosphorylated when combined with KaiC-DE or -DA subunits, which inhibited kinase activity ( Figs 3c and 4a ). 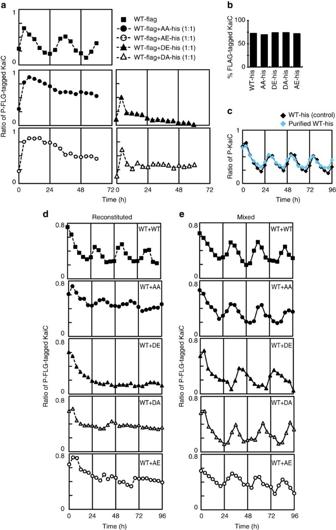Figure 4: Intersubunit interactions are important for robust circadian rhythm. (a) KaiA and KaiB were mixed with reconstituted KaiC hexamers from a 1:1 mixture of monomeric KaiC-WT and mutant KaiC. Aliquots of the reaction mixtures were subjected to western blotting. The ratio of phosphorylated FLAG-tagged KaiC-WT to total FLAG-tagged KaiC-WT was plotted over time. (b) Hexameric KaiC was reconstituted from a 5:1 mixture of FLAG-tagged KaiC-WT and His-tagged KaiC-WT or -mutant monomers. Hexamers containing His-tagged KaiC were collected by Ni-affinity chromatography. Reconstituted hexamers were subjected to immunoblotting using anti-FLAG and anti-His antibodies, and the percentage of FLAG-tagged KaiC-WT in reconstituted hexamers was estimated by densitometric analysis of serial dilutions of standard protein. (c) KaiA and KaiB were mixed with either non-treated His-tagged KaiC-WT hexamers (black line) or His-tagged KaiC-WT hexamers purified by Ni-affinity chromatography (blue line). The ratio of phosphorylated KaiC to total KaiC was plotted against time. (d,e) KaiA and KaiB were mixed with either reconstituted hexamers (d) or a 5:1 mixture of FLAG-tagged KaiC-WT and His-tagged KaiC-mutant hexamers (e). Aliquots were collected and subjected to western blotting and densitometry analysis. The ratio of phosphorylated FLAG-tagged KaiC-WT to total FLAG-tagged KaiC-WT is plotted. Figure 4: Intersubunit interactions are important for robust circadian rhythm. ( a ) KaiA and KaiB were mixed with reconstituted KaiC hexamers from a 1:1 mixture of monomeric KaiC-WT and mutant KaiC. Aliquots of the reaction mixtures were subjected to western blotting. The ratio of phosphorylated FLAG-tagged KaiC-WT to total FLAG-tagged KaiC-WT was plotted over time. ( b ) Hexameric KaiC was reconstituted from a 5:1 mixture of FLAG-tagged KaiC-WT and His-tagged KaiC-WT or -mutant monomers. Hexamers containing His-tagged KaiC were collected by Ni-affinity chromatography. Reconstituted hexamers were subjected to immunoblotting using anti-FLAG and anti-His antibodies, and the percentage of FLAG-tagged KaiC-WT in reconstituted hexamers was estimated by densitometric analysis of serial dilutions of standard protein. ( c ) KaiA and KaiB were mixed with either non-treated His-tagged KaiC-WT hexamers (black line) or His-tagged KaiC-WT hexamers purified by Ni-affinity chromatography (blue line). The ratio of phosphorylated KaiC to total KaiC was plotted against time. ( d , e ) KaiA and KaiB were mixed with either reconstituted hexamers ( d ) or a 5:1 mixture of FLAG-tagged KaiC-WT and His-tagged KaiC-mutant hexamers ( e ). Aliquots were collected and subjected to western blotting and densitometry analysis. The ratio of phosphorylated FLAG-tagged KaiC-WT to total FLAG-tagged KaiC-WT is plotted. Full size image Next, we reconstituted hexamers from a 5:1 mixture of FLAG-tagged KaiC-WT and His-tagged KaiC-AA, -DE, -DA or -AE monomers. As the excess of KaiC-WT made it likely that WT-only hexamer would be abundant in the mixture, hexamers containing His-tagged mutant KaiC were purified by Ni-affinity chromatography ( Supplementary Fig. S12 ). Following purification, WT and mutant KaiC were present in reconstituted hexamers at a ratio of 4–5:1 ( Fig. 4b ). Purified KaiC-WT hexamers exhibited the phosphorylation rhythm of untreated KaiC, indicating that the purification process did not affect KaiC function ( Fig. 4c ). FLAG-tagged KaiC-WT reconstituted with His-tagged KaiC-WT exhibited stable phosphorylation rhythms of normal amplitude; however, the rhythmic change in KaiC-WT phosphorylation was not observed in hexamers reconstituted from FLAG-tagged KaiC-WT and His-tagged KaiC-DE, -DA or -AE. By contrast, FLAG-tagged KaiC-WT reconstituted with His-tagged KaiC-AA exhibited a weak low-amplitude rhythm ( Fig. 4d ), suggesting that the phosphorylation state of a small amount of protomer could influence the whole KaiC hexamer via intersubunit communications, resulting in a robust rhythm. Alternatively, because the affinities of KaiA and KaiB for KaiC are influenced by the phosphorylation state of KaiC [14] , the addition of a phosphorylation mutant to the reaction mixture might change the effective concentrations of KaiA and KaiB, resulting in arrhythmicity. To explore this possibility, we checked the phosphorylation of KaiC-WT in a 5:1 mixture of hexameric KaiC-WT and KaiC-mutant in the presence of KaiA and KaiB. Although KaiC-WT mixed with KaiC-DE hexamer exhibited a slightly altered period, KaiC-WT generally exhibited stable phosphorylation rhythms of normal amplitude in mixtures with mutant hexamers ( Fig. 4e ). Our results reveal the molecular mechanism underlying KaiC’s regulation from the perspective of its hexameric structure. We identified two types of mechanisms for the regulation of KaiC’s autokinase and autophosphatase activities: interactions within interfaces and intersubunit communications. The phosphatase activity was regulated only at reaction units; specifically, the phosphorylation state of one phosphorylation site locally affects its own subunit interfaces and thereby influences dephosphorylation of the adjacent residue ( Fig. 3e ). By contrast, kinase activity was modulated by the phosphorylation state of another protomer in the same hexamer, indicating that it is regulated by intersubunit communications. Our data also demonstrate that the kinase activity of each reaction unit is regulated individually. KaiC-DT exhibited phosphate-incorporation activity similar to that of KaiC-SE ( Supplementary Fig. S5 ). By contrast, the phosphate-incorporation activity of KaiC-WT was decreased by KaiC-DA (corresponding to KaiC-DT) and increased by KaiC-AE (corresponding to KaiC-SE) ( Fig. 3c ). This discrepancy may reflect the existence of two types of regulation of kinase activity. Our findings reveal that the regulatory mechanism of KaiC’s autokinase/autophosphatase activities by phosphorylation state is coupled with ATPase activity and the nucleotide states of the CII domain. KaiC-AAE318Q and KaiC-WT at 4 °C, which are defective in autophosphatase activity, are in the ATP-bound state on CII domain ( Fig. 2 and Supplementary Fig. S6 ), suggesting that normal autophosphatase activity requires ADP binding at the CII domain interface. Contact with nucleotide at the subunit interface might vary according to temperature, resulting in different phosphatase activities at 4 °C and 30 °C. Regarding kinase activity, it is conceivable that structural changes, such as alteration in the distance between phosphorylation sites and γ-phosphate during the ATPase cycle, may directly affect autokinase activity, because CII ATPase-defective mutant KaiC-E318Q lacks autokinase activity though it binds ATP ( Figs 1 and 2 ). We therefore propose that the autokinase and autophosphatase activities of KaiC are modulated by ATPase activity and nucleotide binding at the CII domain. The phosphorylation state of KaiC modulates its ATPase activity ( Fig. 2b ; ref. 7 ). Interestingly, we found that nucleotide-binding state was also modulated by phosphorylation state: KaiC-AA, which mimics unphosphorylated KaiC was predominantly in the ATP-bound form, and KaiC-DE, which mimics phosphorylated KaiC was predominantly in the ADP-bound form ( Fig. 2f ). These results suggest that the modulation of ATPase activity by phosphorylation reflects the nucleotide-binding state. The steady-state ATP binding on KaiC-AA may accelerate ATP hydrolysis, whereas the ADP binding on KaiC-DE would be sufficient to decelerate ATP hydrolysis. Based on all of these observations, we propose the following mechanism for the regulation of KaiC’s autokinase and autophosphatase activities by its phosphorylation state at subunit interfaces ( Fig. 5a ): the phosphorylation state of a single residue affects the ATPase activity and nucleotide binding/release within its own reaction unit at CII domain, regulating phosphatase and kinase activity in a manner that influences phosphorylation and dephosphorylation at adjacent residues. ADP on phosphorylated KaiC, which is probably created by ATP hydrolysis, may promote dephosphorylation. By contrast, bound ATP on unphosphorylated KaiC accompanied by dephosphorylation may promote phosphorylation and ATP hydrolysis. The finding that mutation at either S431 or T432 completely abolishes rhythmicity [13] , [14] indicates that local regulation at each reaction unit contributes to rhythm generation. These observations indicate that autokinase and autophosphatase and ATPase activities are interlocked through phosphorylation and nucleotide-binding states, and this relationship switches the balance between autokinase and autophosphatase activities during the circadian cycle. Quantification of KaiC-bound nucleotides over the phosphorylation cycle will help to elucidate these mechanisms. 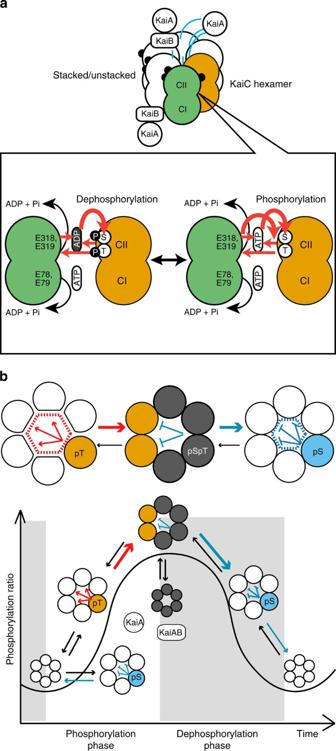Figure 5: Model of the regulatory mechanisms of kinase and phosphatase activities by phosphorylation states. (a) Regulations at subunit interfaces. The CI and CII domains in each protomer of KaiC are represented schematically. CI and CII domains bind ATP or ADP at protomer interfaces. A red line with arrowhead indicates a direction of stimulation effect. (b) Regulation by intersubunit communications. Circles represent KaiC monomers. White, orange, blue and grey represent unphosphorylated (S/T), T432-phosphorylated (S/pT), S431-phosphorylated (pS/T) and double-phosphorylated (pS/pT) states, respectively. Red lines and arrows indicate stimulation of activity. Blue lines and blunt ends represent inhibition of activity. Figure 5: Model of the regulatory mechanisms of kinase and phosphatase activities by phosphorylation states. ( a ) Regulations at subunit interfaces. The CI and CII domains in each protomer of KaiC are represented schematically. CI and CII domains bind ATP or ADP at protomer interfaces. A red line with arrowhead indicates a direction of stimulation effect. ( b ) Regulation by intersubunit communications. Circles represent KaiC monomers. White, orange, blue and grey represent unphosphorylated (S/T), T432-phosphorylated (S/pT), S431-phosphorylated (pS/T) and double-phosphorylated (pS/pT) states, respectively. Red lines and arrows indicate stimulation of activity. Blue lines and blunt ends represent inhibition of activity. Full size image In contrast to the ATPase motif in the CII domain, mutations at catalytic glutamate of CI ATPase (E77QE78Q) did not influence phosphatase or kinase activities ( Fig. 2d–e ); however, the rhythmic change of KaiC phosphorylation was abolished in KaiC-E77QE78Q ( Fig. 2c ; ref. 43 ). Previous work has shown that KaiC-E77QE78Q fails to bind KaiB, resulting in loss of phosphorylation rhythm [43] . Furthermore, CI–CII ring stacking interaction is necessary for KaiBC formation, and KaiB binds to CI [44] . The CI domain may contribute to the regulation of KaiC activity through KaiA and KaiB. It is also possible that KaiC-E77QE78Q has residual CI ATPase activity. Further research is needed to determine whether and how the CI and CII domains interact. In addition, the location of the KaiB-binding site on the KaiC hexamer remains controversial [5] , [44] , [45] , [46] , [47] , [48] . Unambiguous determination of this binding site will help elucidate the molecular mechanisms underlying the regulation of KaiC. Our data provide direct experimental evidence for the functional significance of intersubunit communication within KaiC hexamers and mechanistic insight into how this communication contributes to oscillatory mechanisms ( Figs 3 and 4 ). What, then, is the basis for the molecular mechanisms by which the phosphorylation state of one protomer regulates the kinase activity throughout the whole hexamer? As kinase activity was detected even in reconstituted mixed hexamers composed of unphosphorylated mutant and WT protein ( Fig. 3c ), it is unlikely that phosphorylation in one protomer results in phosphorylation at an adjacent protomer in a stepwise fashion. It is also unlikely that phosphorylation of one protomer affects nucleotide binding of all subunit interfaces, because autophosphatase activity, which was closely related to nucleotide-binding state ( Fig. 2 ), did not change in reconstituted mixed hexamers of WT protein and phosphorylation mutants ( Fig. 3e ). Thus, phosphorylation state of one protomer is likely to modulate some specific features related to kinase activity, for example, the distance between the γ-phosphate of ATP and S431 or T432. One possibility is that intersubunit communications occur via the A-loops of KaiC (residues 487–497). The A-loops exist in a dynamic equilibrium between buried and exposed positions; the latter promote autophosphorylation, whereas the former promote autodephosphorylation [49] . It has been proposed that A-loop exposure repositions ATP closer to the phosphorylation site [49] , and that the dynamic equilibrium of A-loops is created by CII ring flexibility/rigidity, which is influenced by the phosphorylation states themselves [50] . Thus, phosphorylation state of one protomer may affect the flexibility/rigidity of the CII ring, concomitant with a change in A-loop state throughout the whole hexamer, moving CII-bound ATP molecules within phosphoryl-transfer distance of phosphorylation sites. Alternatively, interactions between residues at the subunit interface may contribute to intersubunit communications. Although the X-ray crystal structures of several different phospho-mimics of KaiC are virtually identical [51] , phosphorylation may result in additional interactions between residues at the subunit interface, thereby stabilizing the subunit interface relative to the unphosphorylated form [34] . The influence of phosphorylation states on interactions between adjacent subunits may in turn affect subunit contacts throughout the hexamer, changing the distances between γ-phosphates and phosphorylation sites, including non-adjacent ones. What is the role of intra-hexameric regulation in the circadian mechanism? Our results suggest that intra-hexameric interactions are important for synchronization. Protomers corresponding to KaiC in the phosphorylation phase enhance the kinase activity of other protomers in the same hexamer, resulting in strong hexameric autokinase activity; inversely, protomers corresponding to KaiC in the dephosphorylation phase decrease kinase activity ( Fig. 3 ). Such regulation was observed in the presence of KaiC alone; addition of KaiA increased activity, but did not affect the reaction’s direction ( Fig. 3 ). We also found that even when KaiA and KaiB were added, KaiC-WT was fixed in the phosphorylated form when combined with a protomer that enhanced kinase activity, but fixed in the dephosphorylated form when combined with a protomer that inhibited kinase activity ( Fig. 4a ). These observations suggest that intra-hexameric interactions are important for synchronization, but not generation, of the KaiC phosphorylation rhythm ( Fig. 5b ). Phosphate is incorporated at T432 of a dephosphorylated protomer, resulting in strong hexameric autokinase activity that provides positive feedback that promotes formation of a phosphorylated hexamer. Phosphate is also incorporated onto S431 ( Supplementary Fig. S5 ), but the kinase activities of other protomers are inhibited by S431-phosphorylated KaiC, which is converted back into unphosphorylated KaiC by dephosphorylation. The double-phosphorylated protomer represses autokinase activity in the hexamer. S431-phosphorylated KaiC protomers also repress autokinase activity, preventing re-phosphorylation of T432. This intra-hexameric regulation allows KaiC molecules that were phosphorylated in the wrong order to turn back, while allowing molecules in the appropriate phosphorylation state to move forward in the cycle. As a result, phase coherence among the ensemble of phosphorylating KaiC hexamers is achieved. The weak low-amplitude rhythm with 24-h periodicity in mixed hexamers containing KaiC-WT and KaiC-AA in a 5:1 ratio ( Fig. 4d ) also supports this idea. The KaiC phosphorylation rhythm is robust against changes in concentration of Kai proteins [41] , and persists for 10 days without damping [42] . These observations suggest that in order to sustain robust population-level oscillations, individual KaiC molecules are precisely synchronized to avoid dephasing by the inherent stochasticity of chemical reactions. The simplest assumption that would explain such synchrony is that hexamers can communicate with each other; however, there is no experimental evidence to support such a direct interaction ( Figs 1 and 3 ). The mechanism of synchronization has been the focus of theoretical studies, and two general mechanisms have been proposed: in one, synchronization is achieved by modulation of KaiA and/or KaiB [27] , [29] , [32] , whereas in the other, synchronization is achieved by KaiC via monomer exchange or autocatalysis [25] , [26] , [28] , [52] . In this study, we propose a novel synchronization mechanism, intersubunit communication; however, these mechanisms are not mutually exclusive, and may act together. It is possible that intersubunit communication of kinase activity contributes to the synchronization of phosphorylation phase, and that KaiA sequestration by the KaiBC complex is related to the synchronization of the dephosphorylation phase. We did not detect monomer exchange ( Figs 1 and 3 ); consequently, the results of this study do not reveal any relationship between intersubunit communication and monomer exchange. The circadian clock of an individual cyanobacterial cell is extremely stable [53] , and the resilience of the KaiC phosphorylation rhythm in vitro is thought to reflect the robustness of oscillation in vivo . Robustness of oscillation in the context of molecular noise is a general and important feature of circadian clocks. In eukaryotic circadian systems, the basic timing mechanism is based on transcriptional/translational feedback loops [54] . However, the discovery of a cellular clock in red blood cells and algae [55] , [56] , [57] raises the possibility that eukaryotes might also keep time using metabolic rhythms and biochemical mechanisms similar to those in cyanobacteria. Indeed, many components of the eukaryotic circadian clock have oligomeric structures, and post-translational modifications including phosphorylation are crucial for their activities [58] . Cooperative regulation of clock molecules based on oligomeric structures may be a general feature of the sustained robustness of oscillation in other circadian systems. Moreover, several studies have indicated that ATP binding and hydrolysis of AAA/AAA+ proteins are regulated cooperatively at the intersubunit level [59] , [60] , [61] . Elucidation of the mechanism of KaiC ATPase regulation with regard to intersubunit interactions, and the relationships between the protein’s three activities (ATPase, autokinase and autophosphatase), will be important to advancing our understanding of the principles underlying the circadian clock, as well as the architecture of the regulatory mechanisms of ring-shaped multifunctional enzymes. Purification of recombinant Kai proteins Synechococcus KaiA, KaiB, KaiC and mutant KaiC proteins were expressed in E. coli and purified as previously described [14] . Recombinant GST fusion Kai proteins were produced in E. coli BL21, followed by purification with glutathione-Sepharose beads (GE Healthcare). After removal of the GST tag with the PreScission Protease (GE Healthcare), proteins were further purified by Resource Q anion exchange chromatography (GE Healthcare) and gel-filtration chromatography. Construction of plasmids Mutated kaiC genes encoding E77QE78Q, E318Q, AAE318Q, S431A/T432E and S431D/T432A were constructed by introducing the appropriate mutations into a pGEX6P-1 vector encoding WT KaiC [6] , S431AT432A KaiC [13] or KaiC tagged with a FLAG or His 6 epitope at the C terminus [41] , using the QuikChange Mutagenesis Kit (Stratagene). Primers are described in Supplementary Table S1 . Reconstitution of the KaiC phosphorylation cycle in vitro The reconstitution of the KaiC phosphorylation cycle in vitro was performed as previously described [4] . Briefly, KaiC was incubated at 30 °C with KaiA, KaiB and ATP. The final concentrations of KaiA, KaiB and KaiC were 1.2, 3.5 and 3.5 μM, respectively. Every 4 h, aliquots of the reaction mixture were taken. To separate the phosphorylated forms of KaiC, samples were subjected to SDS–PAGE on a gel of 11% total acrylamide with 0.67% crosslinking factor. KaiC bands were detected between the molecular weights of 35 and 45 kDa on this gel ( Supplementary Fig. S3 ). Tagged KaiC was detected by western blotting using an anti-FLAG (Sigma: A8592, antibody dilution 1:10,000) or anti-His 6 antibody (Roche: 11965085001, antibody dilution 1:1,000). Preparation of 32 P-labelled KaiC hexamers 32 P-labelled KaiC hexamers were obtained using a previously described method [38] . Briefly, KaiC hexamers were incubated on ice for 24 h in buffer (20 mM Tris–HCl (pH 8.0), 150 mM NaCl, 5 mM MgCl 2 and 2 mM DTT) in the presence of 1 mM [γ- 32 P]ATP (12 GBq mmol −1 ). Preparation of KaiC monomers The preparation of KaiC monomers was performed as previously described [38] . Briefly, the reaction mixture was passed through desalting columns to remove ATP, and the samples were incubated at 4 °C for 24 h. KaiC monomer fractions were obtained using gel-filtration chromatography. Immunoprecipitation Immunoprecipitation was performed using Protein G Dynabeads (Invitrogen). Aliquots of the reaction mixture containing 5 μg FLAG-tagged KaiC complexes, buffer (20 mM Tris–HCl (pH 8.0), 150 mM NaCl, 1 mM ATP and 5 mM MgCl 2 ) was added to each sample to a final volume of 750 μl. Samples were treated with Protein G Dynabeads to which monoclonal anti-FLAG M2 antibody (Sigma: F1804) was coupled (0.2 mg ml −1 ). After incubation at room temperature, the beads were washed and FLAG-tagged KaiC complexes were eluted from the beads by incubation with SDS sample buffer. Quantitation of FLAG-tagged KaiC in hexamers Serial dilutions of the standard protein (FLAG-tagged KaiC-WT and His-tagged KaiC-WT) and immunoprecipitated samples were loaded onto the same SDS–polyacrylamide gel (10% precast gel, ATTO) and immunoblotting assays. KaiC bands were detected between the molecular weights of 55 and 70 kDa on this gel ( Supplementary Fig. S3 ). Eluates from the beads were analysed by immunoblotting with anti-FLAG (Sigma: A8592, antibody dilution 1:10,000) and anti-His 6 antibody (Roche: 11965085001, antibody dilution 1:1,000). The intensity of each signal was measured with a densitometer. Comparison of the signal intensity of an immunoprecipitated band with that of a standard protein band enabled an estimate of the amount of KaiC in each eluate. Detection of KaiC-bound nucleotides Nucleotides bound to KaiC were analysed by reconstituting KaiC hexamers from monomers in the presence of 1 mM [α- 32 P]ATP, as previously described [38] . The number of adenine nucleotides bound to each KaiC protomer was nearly constant at 2, indicating that the nucleotide-binding sites of both CI and CII were occupied [38] . Ni-affinity chromatography Purification of His-tagged KaiC was performed using His Mag Sepharose Ni (GE Healthcare). Purified samples were passed through desalting columns equilibrated with buffer (20 mM Tris–HCl (pH 8.0), 150 mM NaCl, 1 mM ATP and 5 mM MgCl 2 ). Autodephosphorylation assay The autodephosphorylation assay was performed as previously described [38] . Briefly, KaiC was labelled with [γ- 32 P]ATP, and the reaction was initiated by removing unincorporated [γ- 32 P]ATP using desalting columns and incubating at 30 °C. Aliquots of the reaction mixture were collected, and the reactions were halted by addition of SDS sample buffer. The resulting samples were subjected to SDS–PAGE. The 32 P-derived signals were detected by autoradiography. KaiA was added at a final concentration of 1.2 μM. KaiC autokinase assay The autokinase assay was performed as previously described [12] with some modifications. KaiC was dephosphorylated by incubation at 30 °C for 24 h. Dephosphorylated KaiC was incubated in a reaction buffer consisting of 20 mM Tris–HCl (pH 8.0), 150 mM NaCl, 1 mM [γ- 32 P]ATP (12.3 GBq mmol −1 ) and 5 mM MgCl 2 . The reactions were halted by addition of SDS sample buffer, and the proteins were separated by SDS–PAGE (10% precast gel, ATTO) and blotted onto PVDF membranes. 32 P-derived signals were detected by autoradiography. Standard curves used to calculate the concentrations of 32 P-labelled molecules from the autoradiograms were generated using serial dilutions of 1 mM [γ- 32 P]ATP (12 GBq mmol −1 ). KaiA was added at a final concentration of 1.2 μM. ATPase measurements ATPase activity of KaiC was measured using an ACQUITY UPLC system (Waters) as described previously [62] . ADP was separated from ATP on a BEH C18 column (Waters) with a mobile phase of 20 mM ammonium phosphate, 10 mM tetrabutylammonium hydrogen sulphate (pH 8.5) and 17% ( v / v ) acetonitrile. The ATPase activity was evaluated as a function of the amount of ADP produced. How to cite this article: Kitayama, Y. et al. KaiC intersubunit communication facilitates robustness of circadian rhythms in cyanobacteria. Nat. Commun. 4:2897 doi: 10.1038/ncomms3897 (2013).